DNA-directed self-assembly of shape-controlled hydrogels Using DNA as programmable, sequence-specific ‘glues’, shape-controlled hydrogel units are self-assembled into prescribed structures. Here we report that aggregates are produced using hydrogel cubes with edge lengths ranging from 30 μm to 1 mm, demonstrating assembly across scales. In a simple one-pot agitation reaction, 25 dimers are constructed in parallel from 50 distinct hydrogel cube species, demonstrating highly multiplexed assembly. Using hydrogel cuboids displaying face-specific DNA glues, diverse structures are achieved in aqueous and in interfacial agitation systems. These include dimers, extended chains and open network structures in an aqueous system, and dimers, chains of fixed length, T-junctions and square shapes in the interfacial system, demonstrating the versatility of the assembly system. Self-assembly is the process by which small components self-organize into larger structures. Initially developed as a concept for engineering molecular complexes [1] , self-assembly has been used to fabricate structures across scales, using monomer units ranging from nanoscale to macroscale dimensions [2] . Diverse techniques have been developed for mesoscale (micrometer to millimeter scale) self-assembly using magnetic force [3] , hydrophile–lipophile balance [4] , [5] , capillary interaction [6] and synthetic chemical binding [7] to control the assembled architecture. Increasing the complexity of mesoscale self-assembly faces a crucial challenge, namely the difficulty of engineering a large set of orthogonal-specific binding interactions between the monomer units. This challenge can be potentially addressed by using DNA, biology’s information carrier, as a programmable ‘glue’ to direct the assembly of mesoscale units. DNA contains four different nucleotide bases, each of which forms a base pair with another complementary base according to a set of canonical rules: adenine with thymine and guanine with cytosine. By simply arranging the sequence of these four nucleotide bases in different DNA strands, a combinatorially large set of binding interactions can be designed as specific hybridizations between complementary DNA strands. DNA hybridization-based self-assembly principles have been utilized successfully in the field of DNA nanotechnology to generate diverse complex synthetic DNA/RNA nanostructures [8] , [9] , [10] , [11] with arbitrarily prescribed geometry [12] , [13] , [14] , [15] , [16] , [17] , [18] , [19] , [20] , [21] , [22] , [23] , [24] , [25] , [26] , [27] , [28] , [29] and dynamic functions [30] , [31] , [32] , [33] , [34] , [35] , [36] , [37] , [38] , [39] , [40] , [41] . Furthermore, DNA strands can be made into hydrogels through covalent [42] , [43] , [44] or non-covalent interactions [45] . DNA has also been used as templates or glues to mediate the self-assembly of fluorophores [46] , proteins [47] , inorganic nanoparticles [48] , [49] , [50] , [51] , carbon nanotube [52] , lipid vesicles [53] and even living cells [54] . Recently, it was reported that short single-stranded DNA probes attached to a glass surface can successfully catch 100 μm size hydrogel microspheres decorated with sequences complementary to the probes [55] . Building on these previous successes, we address the next challenge here: to fully utilize the versatile programmability of DNA to direct the self-assembly of mesoscale objects into complex higher order structures with precisely prescribed architecture and geometry. As part of our work to increase the complexity of the architectural and geometrical control of DNA-directed mesoscale assembly, here, we report on combining DNA-directed assembly principles with microfabrication technology to assemble mesoscale objects using shaped-controlled hydrogel units. The central conceptual innovation here is the decoration of DNA glues onto the prescribed surfaces of a non-spherical hydrogel object to produce an asymmetric glue pattern. These new assembling units, by combining the molecular programmability of the DNA glue and the shape controllability of microfabrication, will provide a powerful platform to achieve programmable assembly of complex mesoscale structures. To implement this strategy, a crucial technical innovation was necessary: we invent a novel strategy to use in situ rolling circle amplification (RCA) to produce and attach ‘giant’ DNA glues to the surface of hydrogel cubes. On the basis of this technical innovation, we demonstrate that giant DNA glue strands, but not short DNA primers, induce the assembly of hydrogel gel cubes with edge lengths across scales (30 μm to 1 mm), and that they result in the self-assembly of cube dimers in a highly multiplexed manner (25 orthogonal dimer pairs from 50 distinct cube species in one pot mixing). We then develop a method to engineer hydrogel cuboids that display giant DNA only on designated faces. Using this technology, we demonstrate the assembly, in aqueous and in interfacial systems, of diverse structures: linear chains with extended or fixed length, open networks, T-junctions and 2 × 2 square structures. Thus, we establish DNA-directed assembly of shape-controlled mesoscale units as a promising route to produce complex structures with sophisticated geometrical and architectural control. Self-assembly of hydrogels with uniform surface DNA glues In the first part of our study, we developed a strategy to use complementary DNA molecules as glue to direct the self-assembly of hydrogel cubes with an edge length of 250 μm. Our initial attempt to assemble such hydrogel cubes carrying short complementary DNA strands (36 nt poly-T linker followed by 20 nt complementary sequences) failed to induce hydrogel assembly ( Fig. 2c ). This failure may be attributed to the rugged surface morphology of the hydrogel, as revealed by scanning electron microscopy (SEM, Fig. 1d ), and the relatively small size and weak binding interactions between short complementary DNA strands. To accommodate for this rugged hydrogel surface, we developed a strategy to decorate hydrogel surface with ‘giant’ single-stranded DNA ( Fig. 1a ). Specifically, in step 1, amine-bearing short DNA strands (brown, 56 nt) were conjugated to PEG–NHS monomers (blue, MW 3,500 Da) using a standard protocol [56] . In step 2, the DNA–PEG–acrylate was mixed with photocrosslinkable poly(ethylene glycol) diacrylate (PEGDA, 4,000 MW) and 0.5 wt% photoinitiator, and exposed to UV under a photomask with 250 × 250 μm square holes. The height of the cubes was controlled using No. 2 microscope cover glass slides (250 μm in thickness) as spacers. Upon UV exposure, 250 × 250 × 250 μm hydrogel cubes uniformly modified with short DNA primers were produced. In step 3, the DNA primers hybridized with complementary, circular DNA templates (produced by circularization of short linear DNA using CircLigase), through a published procedure known as RCA [57] ; the primer was amplified to produce a long strand with repeated sequences complementary to the circular template. In this paper, we call this long single-strand DNA product ‘giant DNA’. 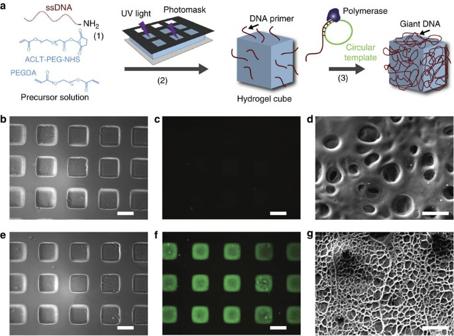Figure 1: Fabrication of hydrogel cubes with uniform giant DNA glue modification. (a) Schematic of the fabrication process of hydrogel cubes uniformly modified with giant DNA. Phase contrast (b,e), fluorescent (c,f) and SEM (d,g) images of hydrogels carrying short 56-nt single-stranded DNA primers (b–d) or amplified single-stranded giant DNA (e–g). The gels incandfwere stained with SYBR Gold before imaging. Scale bar, 200 μm inb,c,eandf; scale bar, 10 μm indandg. Figure 1: Fabrication of hydrogel cubes with uniform giant DNA glue modification. ( a ) Schematic of the fabrication process of hydrogel cubes uniformly modified with giant DNA. Phase contrast ( b , e ), fluorescent ( c , f ) and SEM ( d , g ) images of hydrogels carrying short 56-nt single-stranded DNA primers ( b – d ) or amplified single-stranded giant DNA ( e – g ). The gels in c and f were stained with SYBR Gold before imaging. Scale bar, 200 μm in b , c , e and f ; scale bar, 10 μm in d and g . 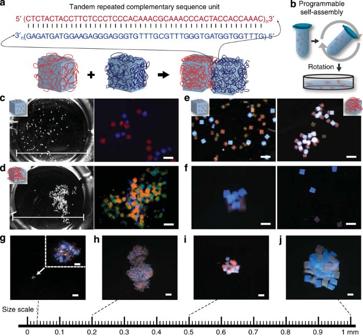Figure 2: Self-assembly of hydrogel cubes with uniform giant DNA glue modification. (a) Schematic of giant-DNA-directed hydrogel assembly. Giant DNA containing tandem repeats of complementary 48-nt sequences was uniformly amplified on the surface of red and blue hydrogel cubes. Hybridization between the complementary DNA sequences resulted in assembly of hydrogel cubes. (b) Hydrogel cubes were assembled in a 0.5ml tube filled with assembly buffer under mild rotation, transferred to a Petri dish with 1.6 cm diameter and imaged under microscope. See Methods for details. (c,d) Phase contrast and fluorescent microscopy images of the post-assembly system, in which hydrogel cubes were modified with short 56-nt (c) or amplified giant (d) DNA strands. Hydrogel cubes carrying complementary DNAaora*were labelled with red or blue fluorescent microbeads, respectively, and stained with SYBR Gold. (e) Red and blue hydrogel cubes carrying complementary short (left) or giant (right) DNA strands failed (left) or succeeded (right) to assemble into aggregates, in the presence of competitive yellow hydrogel cubes that were not modified with DNA. (f) Aggregates assembled from red and blue hydrogel cubes carrying complementary giant DNA fell apart after 1 h Baseline-ZERO DNase treatment (left: before DNase treatment; right: after DNase treatment). Scale bar, 500 μm inc,d,eandf. (g–j) Aggregates were assembled from red and blue hydrogel cubes with various edge lengths: (g) 30 μm, (h) 200 μm, (i) 500 μm and (j) 1 mm. Giant DNA glue was uniformly amplified on the hydrogel surface. Scale bar, 1 mm in the main panels; 50 μm in the inset ofg. Full size image Figure 2: Self-assembly of hydrogel cubes with uniform giant DNA glue modification. ( a ) Schematic of giant-DNA-directed hydrogel assembly. Giant DNA containing tandem repeats of complementary 48-nt sequences was uniformly amplified on the surface of red and blue hydrogel cubes. Hybridization between the complementary DNA sequences resulted in assembly of hydrogel cubes. ( b ) Hydrogel cubes were assembled in a 0.5ml tube filled with assembly buffer under mild rotation, transferred to a Petri dish with 1.6 cm diameter and imaged under microscope. See Methods for details. ( c , d ) Phase contrast and fluorescent microscopy images of the post-assembly system, in which hydrogel cubes were modified with short 56-nt ( c ) or amplified giant ( d ) DNA strands. Hydrogel cubes carrying complementary DNA a or a* were labelled with red or blue fluorescent microbeads, respectively, and stained with SYBR Gold. ( e ) Red and blue hydrogel cubes carrying complementary short (left) or giant (right) DNA strands failed (left) or succeeded (right) to assemble into aggregates, in the presence of competitive yellow hydrogel cubes that were not modified with DNA. ( f ) Aggregates assembled from red and blue hydrogel cubes carrying complementary giant DNA fell apart after 1 h Baseline-ZERO DNase treatment (left: before DNase treatment; right: after DNase treatment). Scale bar, 500 μm in c , d , e and f . ( g – j ) Aggregates were assembled from red and blue hydrogel cubes with various edge lengths: ( g ) 30 μm, ( h ) 200 μm, ( i ) 500 μm and ( j ) 1 mm. Giant DNA glue was uniformly amplified on the hydrogel surface. Scale bar, 1 mm in the main panels; 50 μm in the inset of g . Full size image We first verified the successful production of giant DNA via RCA reaction in free solution and on glass slides ( Supplementary Fig. S2a , agarose gel showed the synthesis of high molecular-weight product; Supplementary Fig. S2b , fluorescent microscopy image showed the formation of large membrane-like giant DNA; Supplementary Fig. S2c , SEM image showed the fiber-like giant DNA on glass slides). We then fabricated hydrogel cubes carrying giant DNA as described above and characterized them using fluorescent DNA staining. In comparison with hydrogels carrying short 56-nt DNA primers ( Fig. 1b , phase contrast imaging; Fig. 1c , fluorescent imaging, DNA was stained by SYBR Gold), 3 h of RCA amplification at 37 °C resulted in significant DNA staining by SYBR Gold ( Fig. 1e , phase contrast imaging; Fig. 1f , fluorescent imaging). As the DNA primer was tethered to the gel precursor, it was anticipated that giant DNA was amplified both inside and on the surface of hydrogel cubes. This is consistent with our experimental observation that only after RCA amplification, the hydrogel cubes stained with fluorescent DNA dye appeared with expected fluorescence under microscope ( Fig. 1c,f ). We note that as the RCA process is diffusion dependent and it is anticipated that it would be diffusion limited in the regions inside the gels relative to the gel surface. It is important that SEM imaging of the gel surface before ( Fig. 1d ) and after ( Fig. 1g ) the RCA amplification provided direct evidence that giant DNA was amplified on the gel surface. After the amplification, the initially rugged surface of the gel was covered uniformly by fiber-like structures, with reduced surface roughness (SEM image, Fig. 1g ). Collectively, the above experiments suggested that the surfaces of hydrogel cubes were decorated with giant DNA produced via RCA, as designed. Next, we demonstrated the giant-DNA-directed assembly of hydrogel cubes. Using the procedure described above, we fabricated 250 × 250 × 250 μm hydrogel cubes carrying giant DNA encoding tandem repeated complementary sequence ( Fig. 2a ), and self-assembly was performed by mixing these hydrogel cubes in a 0.5ml microtube filled with assembly buffer under mild rotation, using a tube rotator with a fixed speed of 18 r.p.m. ( Fig. 2b , see details in Methods). To visualize the assembled structure, the two species of hydrogel cubes carrying complementary DNA sequences a and a * were labelled with red (fluoresbrite microspheres with excitation at 512 nm and emission at 554 nm) or blue (fluoresbrite microspheres with excitation 360 nm and emission 407 nm) fluorescent microbeads, respectively. After the assembly reaction in the tube, the hydrogel cubes were transferred to a 1.6-cm diameter Petri dish for imaging ( Fig. 2b ). Large aggregates were observed for hydrogel cubes carrying complementary giant DNA ( Fig. 2d , left, phase contrast imaging; right, fluorescent imaging). In contrast, hydrogel cubes carrying only 56-nt short DNA primers without RCA amplification failed to produce aggregates under the same assembly conditions ( Fig. 2c , left, phase contrast imaging; right, fluorescent imaging). Including DNA-free yellow hydrogel cubes (that is, cubes that contain yellow microbeads) in the reaction system did not change the assembly outcome for either the hydrogel cubes carrying 56-nt short DNA primers ( Fig. 2e , left) or hydrogel cubes carrying giant DNA ( Fig. 2e , right). Moreover, no yellow hydrogel cubes were observed in the assembled structure, confirming that the assembly was directed by giant DNA on the hydrogel cube surface. This giant-DNA-dependent nature of the assembly was further verified in a DNA-degradation experiment ( Fig. 2f ): assembled hydrogel cubes carrying complementary giant DNA became dispersed after treatment with DNase, which was expected to degrade the giant DNA on the hydrogel cube surface. In previous work, using short DNA strand as glues, researchers were successful in catching small spherical particles (100 μm diameter) on a surface. However, in our system, relatively large cuboid-shaped particles (250 μm edge width) needed to assemble in a strong agitation (to disrupt non-specific interactions) solution-based system, and thus much stronger glue interactions were likely required to enable the assembly. Over 70% specific binding was observed by analyzing the binding event between two hydrogel cubes uniformly carrying same or complementary DNA glues. The giant-DNA-directed hydrogel cube binding was also quantified under different temperatures (4, 25 and 37 °C). We observed that the specific assembly yield increased as the temperature decreased ( Supplementary Fig. S3 ). However, non-specific binding also increased significantly at 4 °C (data not shown). The assembly experiments in the remainder of the paper were performed under room temperature ( Supplementary Fig. S3 ). We next demonstrated that the interaction between complementary giant DNA was capable of directing the assembly of hydrogel cubes with a wide range of edge lengths. Cubes carrying complementary DNA a or a* were labelled with red or blue colour microbeads, respectively. Assembly reaction was performed as described above. Aggregates were observed from hydrogel cubes with edge lengths of 30, 200, 500 and 1,000 μm ( Fig. 2g–j ). These experiments indicate that the hybridization between complementary giant DNA was sufficiently strong to induce the assembly of hydrogel cubes across scales. As complementary DNA molecules hybridize with each other in a sequence-dependent manner, it is possible to generate a large number of specific interactions using giant DNA glues with orthogonal sequences. To test whether such DNA sequence-dependent specificity can be applied in our hydrogel cube self-assembly system, fifty 24-nt DNA sequences were designed to produce 25 pairs of orthogonal-specific interactions ( Fig. 3a ; also see Methods and Supplementary Table S1 for DNA sequences). To visually differentiate distinct cube species under stereomicroscope, coloured microbeads were trapped in the core and periphery parts of the cubic hydrogel ( Fig. 3c , top left corner), and pairwise combinations of 5 colours (red, blue, yellow, black and violet) generated 25 distinct signatures. Following fabrication, giant DNA containing tandem repeated sequence was amplified using RCA reaction on the hydrogel surface as described before. The 25 structures were self-assembled in aqueous assembly system. To avoid forming large aggregates that can trap microgels inside and hence hinder the quantification of specific assembly yields, only one copy for each of the 50 hydrogel species was included in one of five independent experiments ( Fig. 3a ). The assembly was performed using agitation of repeated mild rotation at a fixed speed of 18 r.p.m. and strong hand shaking every 30 min to disrupt non-specific binding. The assembled structures were then transferred to a Petri dish for imaging and quantification. Each of the 25 expected specific dimer structures were all identified ( Fig. 3b,c ). In total, 83 structures were analyzed in five independent experiments: of which about 66% dimerized specifically to their complementary sequence, whereas only 16% formed non-specific dimerized pairs ( Fig. 3d ). These experiments demonstrated that the interaction between giant DNA glue is sequence specific and that highly multiplexed assembly can be achieved using our system. To the best of our knowledge, this system includes more specific interactions than all reported mesoscale self-assembly work. 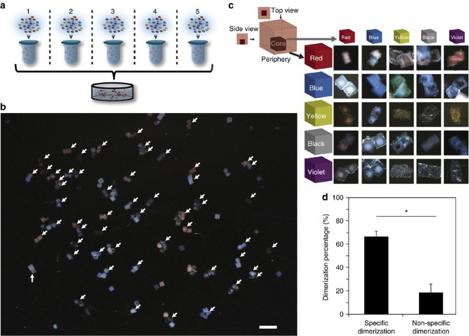Figure 3: Self-assembly of multiple hydrogel cubes dimers. (a) Schematic for multiplexed self-assembly of 25 orthogonal pairs of dimers in five independent experiments. (b) The final assembled structure from five independent experiments were pooled together into a single Petri dish for imaging, and the assembled specific structure was indicated by a white arrow. Scale bar, 1 mm. (c) Schematic (top left) describes the double layer structure of hydrogel cube used in the multiplexed self-assembly of 25 dimers. The core cube was 100 × 100 × 100 μm and the periphery cube was 300 × 300 × 300 μm. See Methods for fabrication details. The core and periphery hydrogel cubes were labelled with distinct coloured microbeads respectively, and pairwise combinations of five colours (red, blue, yellow, black and violet) generated 25 distinct signatures. Images of 25 corresponding dimers are shown. (d) Hydrogel cube dimers were identified under microscopy and quantified as the specific (66±5%) and non-specific (18±7%) binding events,n=5, *P<0.05. Figure 3: Self-assembly of multiple hydrogel cubes dimers. ( a ) Schematic for multiplexed self-assembly of 25 orthogonal pairs of dimers in five independent experiments. ( b ) The final assembled structure from five independent experiments were pooled together into a single Petri dish for imaging, and the assembled specific structure was indicated by a white arrow. Scale bar, 1 mm. ( c ) Schematic (top left) describes the double layer structure of hydrogel cube used in the multiplexed self-assembly of 25 dimers. The core cube was 100 × 100 × 100 μm and the periphery cube was 300 × 300 × 300 μm. See Methods for fabrication details. The core and periphery hydrogel cubes were labelled with distinct coloured microbeads respectively, and pairwise combinations of five colours (red, blue, yellow, black and violet) generated 25 distinct signatures. Images of 25 corresponding dimers are shown. ( d ) Hydrogel cube dimers were identified under microscopy and quantified as the specific (66±5%) and non-specific (18±7%) binding events, n =5, * P <0.05. Full size image Self-assembly of hydrogels with face-specific DNA glues To assemble structures with controlled architecture rather than aggregates, we fabricated hydrogel cuboid units with face-specific giant DNA modification. The procedure is illustrated in Fig. 4a . In steps 1–4, we describe the procedure to make a two-component cube composite structure where a lager ‘body-cube’ displays smaller DNA-modified ‘pad-cubes’ on its designated sides; in steps 5 and 6, we describe the agitation system for their assembly. (Step 1) The 150 × 150 × 150 μm hydrogel pad-cubes were made from a precursor solution that contains 20 wt% PEGDA (4 kDa) and PEG (3.5 kDa) acrylate-ssDNA primers using photolithography. A photomask with 150 × 150 μm square holes was used to control the cross-section shape of the pad-cube; No.1 microscope cover glass slides (150 μm in thickness) were used as spacers to control the height of the pad cube. (Step 2) The unpolymerized reagent was washed away and giant DNA was produced via RCA reaction as described before. We now have arrays of 150-μm pad-cubes (coloured green in Fig. 4a ) with uniform giant DNA modification. (Step 3) To make the larger body-cube, we added a second solution that contained only 20 wt% PEGDA (4 kDa), and covered it with a second photomask with 250 × 250 μm square holes. This photomask was aligned carefully with the pad-cubes made in step 2 such that this photomask covered half of the cross-section area of each pad-cubes (to protect them from subsequent UV exposure). No. 2 microscope cover glass slides (250 μm in thickness) were used as spacers to control the height of the body-cubes. (Step 4) Subsequent UV treatment resulted in the polymerization of the second 250 × 250 × 250 μm body-cube. Unpolymerized reagent was washed away. At the end of step 4, we produced an array of cubes: the red 250 μm body-cube covered half of the green 150 μm pad-cubes; only the green 150 μm pad-cubes were modified with giant DNA. As a consequence, the cube composite only had giant DNA modification on designated faces that display the green pads. For exposition simplicity, we refer to this composite structure as a hydrogel cube with surface-specific DNA modifications. (Step 5) The hydrogel cubes were collected into a 0.5ml microtube filled with the assembly buffer. (Step 6) Assembly was performed by rotating the tube. (Step 7) The solution was transferred to a Petri dish and imaged under microscope. 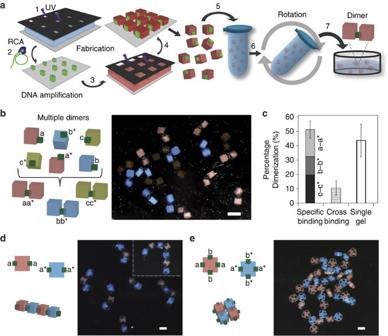Figure 4: Self-assembly of hydrogel cubes with face-specific DNA glue modifications. (a) Hydrogel cubes carrying giant DNA glue on designated faces were fabricated in steps 1–4, collected in a 0.5ml microtube in step 5, mixed and agitated in step 6, and transferred to a Petri dish for imaging in step 7. (b) Hydrogel cubes displaying face-specific giant DNA with tandem repeatsa/a*(with the body cube labelled red),b/b*(blue body cube) orc/c*(yellow body cube). The pad cube carrying giant DNA glue is coloured green. Lettersxandx*denote complementary DNA sequences (seeSupplementary Table S1for sequence details). Scale bar, 500 μm. (c) Quantification of specific assembly, non-specific assembly and unassembled cubes. *P<0.05. (d) Linear chain structures were assembled from the red and blue gels. Left, schematic. Right, microscopy images. The inset shows a chain containing seven cubes. Scale bar, 200 μm. (e) Net-like structures were self-assembled from the red and blue cubes. Scale bar, 200 μm. Figure 4: Self-assembly of hydrogel cubes with face-specific DNA glue modifications. ( a ) Hydrogel cubes carrying giant DNA glue on designated faces were fabricated in steps 1–4, collected in a 0.5ml microtube in step 5, mixed and agitated in step 6, and transferred to a Petri dish for imaging in step 7. ( b ) Hydrogel cubes displaying face-specific giant DNA with tandem repeats a / a* (with the body cube labelled red), b / b* (blue body cube) or c / c* (yellow body cube). The pad cube carrying giant DNA glue is coloured green. Letters x and x* denote complementary DNA sequences (see Supplementary Table S1 for sequence details). Scale bar, 500 μm. ( c ) Quantification of specific assembly, non-specific assembly and unassembled cubes. * P <0.05. ( d ) Linear chain structures were assembled from the red and blue gels. Left, schematic. Right, microscopy images. The inset shows a chain containing seven cubes. Scale bar, 200 μm. ( e ) Net-like structures were self-assembled from the red and blue cubes. Scale bar, 200 μm. Full size image Using the above strategy, we demonstrated the multiplexed assembly of three hydrogel cube dimer species ( Fig. 4b,c ). In this experiment, six hydrogel cube species were manufactured ( Fig. 4b , left). The first species is a red hydrogel cube (that is, the body cube contained red microbeads) that displays giant DNA with tandem repeating sequence ‘ a ’. We call this cube the red cube a. The other five species are red cube a* (where sequence a* is complementary to sequence a ), blue cube b , blue cube b* , yellow cube c and yellow cube c* . Multiple copies of each of the six cube species were made separately and then mixed at room temperature in the same tube for assembly (see Methods for details). After 6-h rotation, the solution was imaged ( Fig. 4b , right). Three populations of the structures were observed and quantified ( Fig. 4c ). In total, 77 assembled structures were analyzed in six independent experiments: 46% were the expected, specific dimers that formed between two same-colour cubes that presumably carried complementary sequences; 10% were the dimers that formed between two different-colour cubes that carried non-complementary sequences; 44% were the unassembled single cubes. The specificity of dimer formation was quantified as 82% by dividing the number of specific dimers over the total number of dimers. Using hydrogel cubes that display giant DNA on multiple designated faces, we next constructed linear chain structures and net-like structures. To make the chain structures, two cube species were made: a red cube that displays giant DNA a on two opposite faces, and a blue cube that displays giant DNA a* on two opposite faces ( Fig. 4d , left). The assembly of these two species produced chain structures that contained alternating red and blue cubes, as expected ( Fig. 4d , right). The longest chain observed contained seven cubes ( Fig. 4d , top-right corner). We then made a red cube species that displays giant DNA a on two opposite faces and giant DNA b on another two opposite faces, and a blue cube species that displays pairs of a* and b* on opposite faces ( Fig. 4e , left). The assembly of these two species resulted in the formation of net-like structures with alternating red and blue cubes that were connected via DNA-modified sides ( Fig. 4e , right). The linear and net-like structures were each assembled in three independent experiments, where each experiment used 40 red and 40 blue complementary cubes. In this experimental system, 39% of the gel cubes remained as unassembled, whereas 58% were assembled into a linear structure (due to their small size, 3% of cubes were lost during the assembly and quantification process). Among the 58% assembled cubes, 42% were only connected to a different colour cube and hence called specifically assembled cubes; the remaining 16% were connected non-specifically to at least one same colour cube, and were called non-specifically assembled cubes. For the net-like structures, the specifically assembled cubes, non-specifically assembled cubes and unassembled cube monomers were, respectively, 56%, 30% and 14%. Interfacial self-assembly of hydrogel to complex structures We next programmed the self-assembly of hydrogel units into prescribed finite structures. To avoid the rotation of the hydrogel cubes in the vertical direction during assembly, flat hydrogel cuboids were fabricated and floated on a liquid/liquid interface between aqueous PBS and Fluorinert FC-40 liquid; horizontal shaking was applied to facilitate assembly ( Fig. 5a ). The assembled structures were directly imaged in this interfacial system. We analyzed the binding between two hydrogel cubes carrying uniform DNA modification in the interfacial system. Over 70% stable specific binding was observed only between hydrogel cubes carrying complementary DNA, which is consistent with what we observed in the aqueous liquid. Using similar fabrication strategy as in Fig. 4a , we made a two-component gel composite: the body is a 1 (length) × 1 (width) × 0.3 mm (height) flat cuboid and the pads are DNA-modified 250 × 250 × 250 μm cubes. Note that the length ratio between the body and the pad cubes increased to 4:1 (as compared with the 1.7:1 in Fig. 4 ). Using the interfacial system and the flat cuboids that carry relatively smaller pads, we were able to assemble dimers ( Fig. 5b ), linear chains with finite length ( Fig. 5c ), a T-junction ( Fig. 5d ) and a square structure ( Fig. 5e ). Note that the linear chain, the T junction and the square are all composed of four distinct cuboid species; by simply changing the pad (and hence surface giant DNA) modification pattern, we were able to change the assembled structure from a chain to a T-junction, and to a square. The assembly process details are captured in time-lapse movies. Supplementary Movie 1 shows two copies of dimers self-assembly ( Fig. 5b ). Supplementary Movie 2 shows the chain structure self-assembly ( Fig. 5c ). Supplementary Movie 3 shows the T-junction self-assembly ( Fig. 5d ). Supplementary Movie 4 shows the self-assembly of the square structures ( Fig. 5e ). 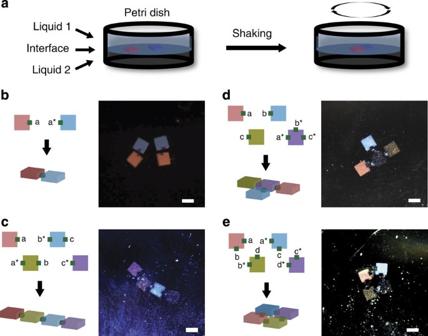Figure 5: Self-assembly of hydrogel cuboids at the liquid–liquid interface. (a) Schematic of hydrogel self-assembly at the liquid–liquid interface. Hydrogel cuboids were floated at the interface formed between upper aqueous PBS liquid and lower Fluorinert FC-40 liquid, and agitated with horizontal shaking. (b) Dimers were formed from the red and blue gels. SeeSupplementary Movie 1for the assembly process. (c–e) Schematic and colour stereomicroscopy images of four hydrogel cuboids (labelled as red, blue, yellow and violet) self-assembled into chain (c) T-junction (d) or square shape (e) based on their surface DNA glue pattern. For the assembly process, seeSupplementary Movies 2, 3 and 4, respectively. Scale bar, 1 mm. Figure 5: Self-assembly of hydrogel cuboids at the liquid–liquid interface. ( a ) Schematic of hydrogel self-assembly at the liquid–liquid interface. Hydrogel cuboids were floated at the interface formed between upper aqueous PBS liquid and lower Fluorinert FC-40 liquid, and agitated with horizontal shaking. ( b ) Dimers were formed from the red and blue gels. See Supplementary Movie 1 for the assembly process. ( c – e ) Schematic and colour stereomicroscopy images of four hydrogel cuboids (labelled as red, blue, yellow and violet) self-assembled into chain ( c ) T-junction ( d ) or square shape ( e ) based on their surface DNA glue pattern. For the assembly process, see Supplementary Movies 2, 3 and 4 , respectively. Scale bar, 1 mm. Full size image For the dimer experiments ( Fig. 5b ), two copies of each component were included; for the linear ( Fig. 5c ), T-junction ( Fig. 5d ) and square ( Fig. 5e ) structures, only one copy of each component was included. We tested the assembly of each system for three times or more, and all together more than 20 experiments were performed for these structures. Out of these more than 20 experiments, the intended structure always formed as desired. However, it is important to note that such systems (involving only one copy of each component) are significantly simpler than systems that involve multiple copies of the same components. We have performed an experiment to form two copies of the T-junction. In this experiment ( Supplementary Fig. S4 ), we started with 14 hydrogel cubes: two copies of centre hydrogel cube (purple) and four copies of each of the three side hydrogel cubes (red, blue and yellow). We attempted the experiments three times, and only successfully assembled two copies of T-junctions in one of the three experiments. It thus remains a challenge to assemble complex structures using multiple copies for each component in the interfacial systems. Although short DNA primer has been reported to assemble nano-particles and microscale hydrogels, we demonstrate, for the first time, the DNA-directed self-assembly of shape-controlled hydrogel modules to build complex structures in a programmable fashion. Acting like sequence-specific glue and tethered onto a microgel surface, giant single-stranded DNA exhibits a significant capability for binding objects across scales, with sizes ranging from 30 micrometers to a millimeter. In addition, giant DNA glues offer significant diversity over current mesoscale self-assembly systems: 50 DNA sequences were designed to generate 25 orthogonal pairs of specific interactions. This is the largest of number of orthogonal-binding interactions that have been used simultaneously in the same reaction system for mesoscale assembly. The designable DNA glues thus provide much richer options for programming mesoscale self-assembly. For self-assembling complex structures, the unit fabrication is crucial. As cube units uniformly carrying DNA glues assembled only into aggregates lack of architecture control, we developed a precisely controlled fabrication technique by which specific giant DNA glue is decorated on a prescribed face of a hydrogel cuboid. By changing the position of DNA glues, various structures including dimers, linear chains and open networks were assembled. In an interfacial system, we further demonstrated that hydrogel cuboids can be fabricated with four different DNA glues on four designated faces, and by simply changing the surface DNA decoration pattern, we assembled discrete structures including dimers, T-junctions, linear chains with fixed length and squares. We have successfully introduced programmability into self-assembling mesoscale structures. We believe that there is still room for improvement in our self-assembly system. For example, it is possible to improve the assembly by tuning the strength of DNA glue through controlling the DNA density and length on the gel surface. In addition, better face-to-face alignment could be achieved by improving the gel fabrication method, for example, by minimizing the aspect ratio between the DNA carrying pads and the gel body (note that the assembly in Fig. 5 demonstrated improved face-to-face alignment over Fig. 4 ). Furthermore, advances in the mixing regimes that better regulate the hydrodynamic forces involved in the assembly process may be used to further enhance the assembly process. By coupling novel in situ DNA amplification methods and microfabrication techniques, we successfully introduced the diversity and specificity of biomolecular interaction to mesoscale assembly. DNA-directed self-assembly of shape-controlled hydrogel modules proved to be highly programmable and controllable, and will open new doors to address the challenge of building complex self-assembled three-dimensional structures for diverse applications in materials science and especially in biomaterials. One particularly promising direction is to develop tissue engineering application, as recreating the highly defined complicate structure of tissue is a pressing challenge. For example, by encapsulating specific cells inside the hydrogel cubes, the self-assembled structures could be used to build the basic architectures of native tissues. Materials The pre-polymer solution of PEGDA with average molecular weight 4,000 Da was prepared by diluting PEG (Monomer-Polymer & Dajac Labs) in DPBS (Gibco) to a final concentration of 20 wt% with 0.5 wt% photo-initiator, 1-(4-(2-Hydroxyethoxy)-phenyl)-2-hydroxy-2-methyl-1-propane-1-one (IRGACURE 2959 Ciba) for hydrogel modules fabrication. A circular DNA template was produced by ligating 5′ and 3′ ends of DNA (Invitrogen) with 5′ end phosphate modification using a CircLigase ssDNA ligase (EPICENTRE Biotechnology). DNA sequence for DNA glue synthesis was designed using software NUPACK ( www.nupack.org ) to minimize mis-hybridization between orthogonal sequences. DNA was ordered from Invitrogen. The baseline-ZERO DNase was obtained from Epicentre Biotechnology and used with final concentration of 1 U ml −1 . Sequence design We designed 25 orthogonal sequence pairs using a modified version of the Domain Design software described by Zhang et al . [58] We first designed 25 domains of 24 bases each, and then concatenated these domains together into 25 domains of 48 bases each. Sequences were designed using a three-letter alphabet to reduce spurious hybridization. To reduce long regions of repeated bases (for example, poly-A, poly-G, and so on), we assign a higher reward to sequences with a higher Shannon entropy. Using NUPACK thermodynamic analysis package, unintended interactions between the concatenated products were calculated to be ~10 8 times less favourable than the intended interactions [59] . Fabrication of PEG hydrogels carrying DNA glues We followed a standard protocol to synthesize acrylate–PEG–DNA by adopting NHS chemistry to conjugate a 5′ amine-modified DNA strand (containing a poly(T-36) linker segment followed by a primer segment) to acrylate–PEG–NHS (Jenkem Technology). Shape-controlled PEG hydrogel was fabricated by following a general photolithograph process as described in our previous work [60] , in which the photomask was designed using AutoCAD software with 200,000 dpi resolution (CAD/Art Services; Bandon, OR). Before DNA amplification, hydrogel was washed with PBS and DNA amplification buffer thoroughly (40 mM Tris–HCl pH 7.5, 50 mM KCl, 10 mM MgCl 2 , 5 mM (NH 4 ) 2 SO 4 , and 4 mM dithiothreitol). Giant DNA was amplified by soaking hydrogel in reaction solution containing 50 μM circular DNA template and 5 U μl −1 of Phi29 DNA polymerase (EPICENTRE Biotechnology) in 1 × DNA amplification buffer at 37 °C overnight according to the manufacturer’s instructions. Hydrogel carrying patterned DNA glue was fabricated in a two-step fabrication process. In step 1, DNA glue was amplified on a small hydrogel cube with edge width of 150–300 μm, which was fabricated by photolithography as described above. In step 2, DNA gel was washed with 1 × assembly buffer (0.5 M NaCl, 0.5 mM EDTA and 0.05% Tween-20 in 1 × PBS) thoroughly. Then 20 wt% pre-polymer PEG solution containing 1 v/v% colour microbead was added. The final shape of hydrogel was controlled by a secondary photomask which was aligned under microscope with the hydrogel to produce the desired DNA pattern. Self-assembly of hydrogels in aqueous solution Hydrogels carrying specific DNA glue was collected in a 0.5ml microtube filled with assembly buffer containing 0.5 M NaCl, 0.5 mM EDTA and 0.05% Tween-20 in 1 × PBS buffer. To prevent non-specific binding between hydrogel and microtube, the inside surface of microtube was treated with a corona treater (BD-20AC from Electro-Technic Products Inc.) and then coated with 10% PEGDA (MW 1,000) beforehand. To achieve DNA-directed hydrogel assembly, microtube was subjected to agitation of continuous 360° upright rotation on a VWR Multimix tube rotator with a fixed speed of 18 r.p.m. and intermittent soft vortex or hand shaking every 30–60 min to disrupt non-specific binding or aggregates at room temperature. After assembly, hydrogel was transferred to a Petri dish filled with a solution of 20 wt% PEG (MW 3,350) in 1 × assembly buffer and subjected to further horizontal shaking at a speed of about 60 r.p.m. on a VWR standard orbital shaker. Assembled structures were identified, quantified and imaged using a Stereo Microscope. Liquid/liquid interface self-assembly Liquid/liquid interface was generated between Fluorinert electronic liquid FC-40 (bottom liquid, 3M Chemicals) and aqueous assembly buffer (top liquid) in a Petri dish. Hydrogel units were floated on the interface and subjected to agitation of continuous horizontal shaking at a low speed of 60 r.p.m. on a VWR standard orbital shaker (Model 1000, VWR) and intermittent 120 r.p.m. shaking or strong hand shaking every 30–60 min to break undesired, spurious aggregates at room temperature. Assembly process was recorded using an image recording software, HyperCam Version 2, under a Stereo Microscope. Quantification of DNA-directed hydrogel assembly To quantify the specificity of dimer formation, hydrogel cubes with an edge width of 250 μm were fabricated. A gel is uniformly decorated with a particular giant DNA glue species. In total, three different complementary pairs of DNA ( a/a *, red; b/b *, blue; c/c *, yellow) were used to generate giant DNA glues. Ten copies of hydrogels of each pair were placed in an Eppendorf tube ( n =6) filled with assembly buffer and rotated for over 3 h. Rotating the hydrogels generated dimers with all different combinations of the three colours. Self-assembly was performed in aqueous liquid system as described above, and the total specific binding among the pairs was identified under a Stereo Microscope. Quantification analysis was performed using STDEV function and TDIST function for s.d. and P -value, respectively, in software Excel (Microsoft). Giant DNA analysis Giant DNA was amplified by RCA using Phi29 DNA polymerase (EPICENTRE Biotechnology), as described earlier and analyzed on a 1% agarose gel with SYBR Green staining. The morphology of giant DNA on surface of microgel or glass slide was analyzed using a SEM (Ziess EVO SEM). After amplification, microgel was rinsed with PBS (GIBCO, DPBS) thoroughly and the liquid around the gel was dried up using Kimwipes. Following washing, microgel was frozen in −80 °C freezer for 3 h and transferred to a freeze drier for 2 days before SEM imaging. Assembly of 25 orthogonal pairs of hydrogel dimmers DNA strands, D001 , D001 *, D002 , D002 * …… D025 , D025 * ( Supplementary Table S1 :DNA sequences), and poly(T-36) with a 5′ end amine modification were purchased from Integrated DNA Technology and dissolved in water upon arrival. DNA oligo phosphorylation One phosphate group was added to the 3′ end of DNA strands by T4 polynucleotide kinase (PNK, EPICENTRE Biotechnology) before ligation with poly(T-36) or circularization. Phosphorylation master reaction containing 33 mM Tris–HCl (pH 7.5), 66 mM potassium acetate, 10 mM magnesium acetate, 0.5 mM dithiothreitol, 5 mM ATP, 100 μM DNA oligo and 10 U μl −1 PNK enzyme was incubated at 37 °C for 3 h and then PNK enzyme was inactivated by incubation at 70 °C for 30 min. Circular DNA template preparation Circular DNA template was prepared by circulating phosphate-modified DNA strand using Cirligase II ssDNA ligase (EPICENTRE Biotechnology). Circularization reaction was performed by supplementing 2.5 mM manganese chloride, 1 M Betaine and 5 U μl −1 ligase to phosphate-modified DNA strand solution and then incubated at 60 °C for 6 h. Then the ligase was inactivated at 80 °C for 10 min. Then exonuclease I (EPICENTRE Biotechnology) was added to remove linear DNA at 37 °C for 1 h and was inactivated at 80 °C for 30 min. Conjugation of acrylate–PEG–DNA primer First, phosphorylated DNA oligo was ligated to amine-poly(T-36). Ligation reaction was performed with supplementing 20 U μl −1 T4 RNA ligase (New England Biolab) and 100 μM amine-poly(T-36) in phosphate-modified DNA oligo solution and incubated at room temperature (25 °C) overnight. Following ligation, amine-poly(T-36)-DNA oligo was conjugated with acrylate-PEG-NHS (Jenkem Technology) as described earlier. Cubic PEG microgel with size of 250 × 250 × 250 μm carrying DNA primer was fabricated, and giant DNA was amplified as described earlier. Pairwise combination of the core and periphery gels that contain one of the five colour microbeads (polybead Red Dyed 1.0-μm microspheres, polybead Blue Dyed 0.5-μm microspheres, Polybead Yellow Dyed 3.0-μm microspheres, polybead Violet Dyed 1.0-μm microsphere and polybead Black Dyed 10.0-μm microspheres; Polysciences) generated 25 distinct labelling. Fabrication process is similar to that of microgel for dimer assembly as previously described except for the following modification. During the secondary photolithography, the second microgel (periphery) was fabricated to completely wrap the first microgel (core) to form the final structure. To decrease assembly time and avoid aggregation, a single copy of each microgel uniformly carrying DNA D001 , D001 *, D002 , D002 * …… D025 , D025 * was collected in 0.5ml Eppendorf microtubes filled with 1 × assembly buffer. Subsequent self-assembly was performed in aqueous liquid as described earlier. The assembled structure was identified under a Stereo Microscope. How to cite this article: Qi, H. et al. DNA-directed self-assembly of shape-controlled hydrogels. Nat. Commun. 4:2275 doi: 10.1038/ncomms3275 (2013).